Bifurcation of the endocytic pathway into Rab5-dependent and -independent transport to the vacuole The yeast Rab5 homologue, Vps21p, is known to be involved both in the vacuolar protein sorting (VPS) pathway from the trans-Golgi network to the vacuole, and in the endocytic pathway from the plasma membrane to the vacuole. However, the intracellular location at which these two pathways converge remains unclear. In addition, the endocytic pathway is not completely blocked in yeast cells lacking all Rab5 genes, suggesting the existence of an unidentified route that bypasses the Rab5-dependent endocytic pathway. Here we show that convergence of the endocytic and VPS pathways occurs upstream of the requirement for Vps21p in these pathways. We also identify a previously unidentified endocytic pathway mediated by the AP-3 complex. Importantly, the AP-3-mediated pathway appears mostly intact in Rab5 -disrupted cells, and thus works as an alternative route to the vacuole/lysosome. We propose that the endocytic traffic branches into two routes to reach the vacuole: a Rab5-dependent VPS pathway and a Rab5-independent AP-3-mediated pathway. Endocytosis is a process in which a portion of the plasma membrane buds inwards towards the cytoplasm to form a clathrin-coated vesicle containing various cargo, such as membrane proteins and extracellular molecules. Once the endocytic vesicles are uncoated, they are capable of fusing with internal organelles, thereby delivering the cargo to the early endosome, where they are sorted to recycling endosomes that bring the cargo back to the plasma membrane [1] , [2] , or to late endosomes/multivesicular bodies (MVBs) en route to the lysosome/vacuole for degradation. Genetic analyses in yeast have led to the identification of over 70 proteins necessary for the transport and sorting of newly synthesized proteins to the yeast vacuole, an organelle that shares several characteristics with the lysosomes of higher animals [3] . These proteins control two major trafficking pathways from the trans-Golgi network (TGN) to the vacuole, the vacuolar protein sorting (VPS) and the adaptor protein (AP)-3-mediated sorting pathways [4] , [5] , [6] . Proteins trafficked via the VPS pathway transit through late endosomes/MVBs en route to the vacuole, whereas the AP-3 pathway mediates transport to the vacuole independently of the late endosomes/MVBs. Although several studies suggested that the route taken to the vacuole by proteins that have been endocytosed from the plasma membrane converges with the route taken by vacuolar proteins traversing the VPS pathway at the late endosomes/MVBs [7] , [8] , [9] , [10] , [11] , the intracellular location at which these pathways converge is still controversial. In addition, the involvement of the AP-3 pathway in the endocytic pathway has not been clear, although several studies suggested a role for AP-3 complex at the early endocytic compartment [12] , [13] . The small GTPase, Rab5, is a key regulator of early endocytosis, being involved in targeting plasma membrane-derived endocytic vesicles to endosomes, fusion between early endosomes, MVB biogenesis and endosomal motility [14] , [15] , [16] , [17] , [18] . In addition to these traditional roles, it has recently been demonstrated that Rab5 has a role in maturation of the early to the late endosome [19] , [20] , [21] . Deletion of the yeast Rab5 gene, VPS21, results in accumulation of the vacuolar protein Vph1p delivered from the VPS pathway and the cell surface receptor, Ste3p, delivered from the endocytic pathway in distinct vesicles [11] , suggesting that Vps21p can function at two distinct transport steps—vacuolar transport from the TGN and the early-to-late endosome transition, before convergence of the endocytic and VPS pathways. Since the specific role of mammalian Rab5 in trafficking from the Golgi to the lysosome has not been well defined, it is difficult to integrate data pertaining to the function of Vps21p in the VPS pathway in yeast with the established roles of mammalian Rab5 in the endocytic pathway. Furthermore, it remains unclear if Rab5 coordinates these two pathways individually and whether Rab5 is necessary for convergence of these pathways. Importantly, the endocytic pathway is not completely blocked in cells lacking all Rab5 genes, including VPS21 , YPT52 and YPT53 , in yeast [22] , suggesting the existence of an unidentified route that can mediate the endocytic pathway instead of the VPS pathway. Unlike other trafficking pathways, the endocytic pathway has an advantage in that the starting compartment, the plasma membrane, is accessible from the extracellular space, and thereby can be visualized using fluorescent molecules that are introduced to the cell externally. We have previously developed fluorescently labelled derivatives of α-factor as novel endocytic markers that bind to the Ste2 receptor, and then become internalized by receptor-mediated endocytosis, finally undergoing trafficking to the vacuole [23] . These fluorescent molecules label the endocytic pathway specifically and time dependently, and do not label other pathways such as the recycling pathway, thereby allowing visualization of the whole route taken by endocytosed cargo before delivery to the vacuole. In the present study, we use these markers to reveal that Vps21p is required for the process of endosome fusion in the Rab5-dependent endocytic pathway. We also identify a Rab5-independent endocytic pathway in yeast that depends on the AP-3 adaptor complex. Subcellular localization of Vps21p in the endocytic pathway Vps21p has been demonstrated to associate with, and regulate, membrane trafficking through late endosomes/MVBs that receive both newly endocytosed cargo as well as newly synthesized proteins that are targeted to the vacuole [11] , [22] . However, the precise step or steps controlled by Vps21p remain unclear. As a first step to clarifying this, we wished to determine its subcellular localization, using an N-terminal GFP-tagged protein expressed from the endogenous locus ( Supplementary Fig. 1a ) (see Methods for details). The functionality of this GFP-tagged Vps21p was confirmed by testing its ability to complement the growth phenotype of vps21 Δ ypt52 Δ cells on YPD plates containing 400 mM CaCl 2 (ref. 18) [18] ( Fig. 1a ). GFP-Vps21p was clearly detected as numerous small puncta throughout the cytoplasm and prevacuolar compartments (PVCs) ( Fig. 1b ). By comparing the localization of GFP-Vps21p with mCherry-tagged specific markers for organelles, we detected high colocalization of GFP-Vps21p with mCherry-tagged Hse1p (79.7±2.3%, mean±s.d., n =3), a marker of the ESCRT-0 complex [24] , [25] , partial colocalization with Vps26p (52.8±10.5%, n =3), a component of the retromer complex that localizes to the late endosomal/PVCs [25] , [26] , and slight colocalization with Sec7p (9.5±2.3%, n =3), a trans-Golgi marker [27] ( Fig. 1c,d ). On the other hand, Vps21p was rarely colocalized with the mitochondria labelled by mitotracker (<2%) used as a negative control ( Fig. 1c,d ). We next utilized Alexa Fluor 594-α-factor (A594-α-factor), to label the receptor-mediated endocytic pathway [23] , [28] and examine the localization of Vps21p in endocytic compartments. GFP-Vps21p was highly colocalized with A594-α-factor-labelled endosomes at 5–10 min after α-factor internalization ( Fig. 1e,f ). In contrast, little localization of Alexa Fluor 488-α-factor (A488-α-factor) was observed in the mitochondria (<2%) ( Fig. 1e ). These data show that the predominant localization of Vps21p is at early-to-late endosomes. Notably, within 5 min after A594-α-factor internalization, we often observed endosomes, colabeled with A594-α-factor and GFP-Vps21p, fusing with each other and resulting in the formation of enlarged endosomes ( Fig. 1g and Supplementary Movie 1 ). These observations suggest that Vps21p is localized to maturing endosomes and might mediate fusion of these compartments. 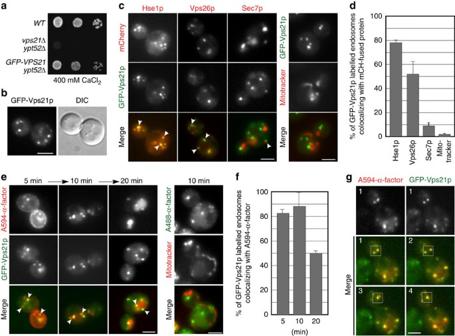Figure 1: Localization of GFP-tagged Vps21p expressed from its endogenous promoter in the endocytic pathway. (a) GFP-Vps21p complemented the growth phenotype ofvps21Δypt52Δ cells. A dilution series of cells was plated on yeast extract peptone-dextrose (YPD) plates containing 400 mM CaCl2and incubated at 25 °C. (b) The endogenous localization of GFP-Vps21p in living cells. Cells expressing GFP-Vps21p were grown to early to mid-logarithmic phase in YPD medium at 25 °C and observed by fluorescence microscopy and different interference contrast (DIC). (c) Localization of GFP-Vps21p and mCherry-tagged organelle markers in wild-type cells. Each image pair was acquired simultaneously using dual-channel two-dimensional (2D) imaging system (see Methods for details). Merged images of GFP and mCherry channels are shown in the lower panel. Arrowheads indicate examples of colocalization. (d) Quantification of colocalization of GFP-Vps21p and mCherry-tagged organelle markers. Colocalization was defined by the presence of two fluorescence molecules at the same location in single focal plane images. The percentages of colocalization were calculated as the ratio of GFP-Vps21p-labelled endosomes (n=100) colocalizing with each marker in each experiment. Error bars indicate the s.d. from at least three independent experiments. (e) Localization of GFP-Vps21p in endocytic compartments. Cells expressing GFP-Vps21p were labelled with A594-α-factor as described in Methods. The images were acquired simultaneously at 5, 10 and 20 min after washing out unbound A594-α-factor and warming the cells to 25 °C. Right panels show localization of A488-α-factor and mitotracker in wild-type cell. (f) Quantification of the colocalization of GFP-Vps21p with A594-α-factor at each time point. Colocalization was defined as described in (d). The percentages of colocalization were calculated as the ratio of A594-α-factor localized in Vps21p-positive compartments (n=50) in each experiment. Error bars represent the s.d. from at least three experiments. (g) Fusion of endosomes containing GFP-Vps21p and A594-α-factor (Supplementary Movie 1). Endosomes labelled with GFP-Vps21p and A594-α-factor were imaged in wild-type cells. Boxed areas denote the sites where two independent endosomes co-labelled with GFP-Vps21p and A594-α-factor were fused with each other, resulting in the formation of enlarged endosome. Time to acquire one image pair was 3.0 s. Scale bars, 2.5 μm. Figure 1: Localization of GFP-tagged Vps21p expressed from its endogenous promoter in the endocytic pathway. ( a ) GFP-Vps21p complemented the growth phenotype of vps21 Δ ypt52 Δ cells. A dilution series of cells was plated on yeast extract peptone-dextrose (YPD) plates containing 400 mM CaCl 2 and incubated at 25 °C. ( b ) The endogenous localization of GFP-Vps21p in living cells. Cells expressing GFP-Vps21p were grown to early to mid-logarithmic phase in YPD medium at 25 °C and observed by fluorescence microscopy and different interference contrast (DIC). ( c ) Localization of GFP-Vps21p and mCherry-tagged organelle markers in wild-type cells. Each image pair was acquired simultaneously using dual-channel two-dimensional (2D) imaging system (see Methods for details). Merged images of GFP and mCherry channels are shown in the lower panel. Arrowheads indicate examples of colocalization. ( d ) Quantification of colocalization of GFP-Vps21p and mCherry-tagged organelle markers. Colocalization was defined by the presence of two fluorescence molecules at the same location in single focal plane images. The percentages of colocalization were calculated as the ratio of GFP-Vps21p-labelled endosomes ( n =100) colocalizing with each marker in each experiment. Error bars indicate the s.d. from at least three independent experiments. ( e ) Localization of GFP-Vps21p in endocytic compartments. Cells expressing GFP-Vps21p were labelled with A594-α-factor as described in Methods. The images were acquired simultaneously at 5, 10 and 20 min after washing out unbound A594-α-factor and warming the cells to 25 °C. Right panels show localization of A488-α-factor and mitotracker in wild-type cell. ( f ) Quantification of the colocalization of GFP-Vps21p with A594-α-factor at each time point. Colocalization was defined as described in ( d ). The percentages of colocalization were calculated as the ratio of A594-α-factor localized in Vps21p-positive compartments ( n =50) in each experiment. Error bars represent the s.d. from at least three experiments. ( g ) Fusion of endosomes containing GFP-Vps21p and A594-α-factor ( Supplementary Movie 1 ). Endosomes labelled with GFP-Vps21p and A594-α-factor were imaged in wild-type cells. Boxed areas denote the sites where two independent endosomes co-labelled with GFP-Vps21p and A594-α-factor were fused with each other, resulting in the formation of enlarged endosome. Time to acquire one image pair was 3.0 s. Scale bars, 2.5 μm. Full size image Fusion of early endosomes is impaired in vps21 Δ ypt52 Δ cells To clarify the step(s) of endocytic transport that require the function of Vps21p, we examined the effect of deleting VPS21 family genes on the endocytic pathway. We first confirmed that deletion of the VPS21 gene had little effect on 35 S-labelled α-factor internalization even when combined with ypt52 Δ, suggesting that Vps21p and Ypt52p are not required for the formation and internalization of endocytic vesicles [22] ( Supplementary Fig. 1b ). We next labelled wild-type and VPS21 family mutant cells with A594-α-factor and followed the localization at several time points after α-factor internalization. Aberrant accumulation of A594-α-factor in multiple endosomal compartments was observed in vps21 Δ cells, resulting in a delay of α-factor transport to the vacuole ( Fig. 2a ). In contrast, single mutants for YPT52 or YPT53, another paralog of VPS21 , showed only a negligible defect in A594-α-factor transport ( Fig. 2b ), consistent with a prior study [22] . Quantitative analysis categorizing A594-α-factor localization as vacuole only, endosome and vacuole or endosome only, revealed that the combination of the vps21 Δ and ypt52 Δ mutations had a more severe effect than the vps21 Δ single mutants ( Fig. 2a,b ). No further additional effect was observed in vps21 Δ ypt52 Δ ypt53 Δ triple mutants. We next analysed temporal changes in the number of A594-α-factor-positive endosomes. A594-α-factor began to accumulate in the early endocytic compartments, resulting in an increased number of A594-α-factor-labelled endosomes, by 5 min in both wild-type and vps21 Δ ypt52 Δ cells ( Fig. 2c,d ). In wild-type cells, after reaching a maximum, the number of A594-α-factor-labelled endosomes decreased until most A594-α-factor had been transported to the vacuole ( Fig. 2c,d ). In contrast, the number of endosomes in vps21 Δ ypt52 Δ cells increased continuously until 10 min after α-factor internalization, and reached about a threefold higher level than that seen in wild-type cells ( Fig. 2c,d ). The behaviours of A594-α-factor-labelled endosomes in vps21 Δ ypt52 Δ cells were not affected by expressing GFP-fused proteins used in this study ( Supplementary Fig. 2 and Supplementary Movie 2 ). These observations suggest that progression beyond the early endocytic stage is impaired in vps21 Δ ypt52 Δ cells. Next, using electron microscopy, we explored the ultrastructure of endosomal compartments where α-factor had accumulated. Various sizes of accumulated vesicles (~40–150 nm) were observed in vps21 Δ ypt52 Δ cells, whereas in wild-type cells such structures were rarely detected ( Fig. 2e ). The range of vesicle diameters was relatively greater than that of vesicles identified previously (~40–60 nm) [22] . To identify the endosomal compartment in which α-factor had accumulated at a higher level of resolution, we used immuno-EM. When applied to wild-type cells, the anti-Alexa Fluor 488 antibody predominantly labelled the vacuole ( Fig. 2f ). In contrast, vps21 Δ ypt52 Δ cells showed several clusters of gold particles over vesicles of different sizes ( Fig. 2f ). Their diameter of ~40–150 nm supported the conclusion that these are endosomes rather than endocytic vesicles. Thus our analysis supports the idea that transport of α-factor is inhibited at the early endosome stage in vps21 Δ ypt52 Δ cells due to a block in endosomal fusion and maturation. 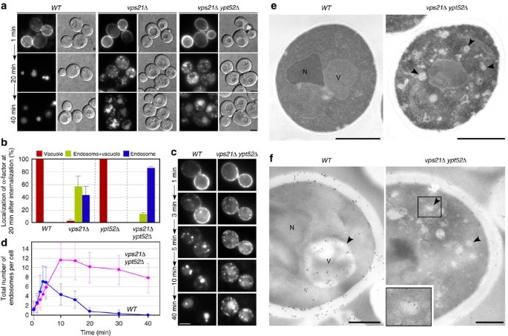Figure 2: Accumulation of A594-α-factor in increased and enlarged endosomes invps21Δypt52Δ cells. (a) Defective transport of A594-α-factor invps21Δ cells. Wild-type,vps21Δ orvps21Δypt52Δ cells were treated with A594-α-factor, and the images were acquired 1, 20 and 40 min after washing out unbound A594-α-factor and warming the cell to 25 °C. Scale bars, 5 μm. (b) Quantification of localization of A594-α-factor in wild-type and mutant cells at 20 min after internalization. Localization of A594-α-factor was categorized into three classes; vacuole only (red), endosome and vacuole (green) and endosome only (blue). Data show mean±s.d. from at least three experiments, with >100 cells counted for each strain per experiment. (c) Time-dependent changes of A594-α-factor localization in wild-type andvps21Δypt52Δ cells. Wild-type andvps21Δypt52Δ cells were labelled with A594-α-factor and imaged at indicated times. Scale bars, 2.5 μm. (d) Quantification of the number of A594-α-factor-positive endosomes displayed in (c). Data show the mean±s.d. of three experiments, with 50 cells counted at each time point per experiment. (e) Ultrastructure of endosomal compartments observed in wild-type andvps21Δypt52Δ cells. Wild-type andvps21Δypt52Δ cells were grown at 25 °C, and fixed with 2% formaldehyde and 2.5% glutaraldehyde in phosphate buffer. Arrowheads point to various sizes of vesicles that accumulate invps21Δypt52Δ cells. V, vacuole; N, nucleus. Scale bars, 1 μm. (f) Immunoelectron microscopic localization of A488-α-factor in wild-type andvps21Δypt52Δ cells. Wild-type andvps21Δypt52Δ cells were incubated with A488-α-factor and internalization was induced 20 min before 4% formaldehyde/0.05% glutaraldehyde fixation. Internalized A488-α-factor was labelled with rabbit anti-Alexa Fluor 488 antibody followed by biotinylated goat anti-rabbit immunoglobulin G and then goat anti-biotin immunoglobulin G-CG (8 nm) conjugate. The bottom panel invps21Δypt52Δ cell shows a high-magnification view of the boxed area. Arrowheads point to vesicular structures including A488-α-factor. Scale bars, 500 nm. Figure 2: Accumulation of A594-α-factor in increased and enlarged endosomes in vps21 Δ ypt52 Δ cells. ( a ) Defective transport of A594-α-factor in vps21 Δ cells. Wild-type, vps21 Δ or vps21 Δ ypt52 Δ cells were treated with A594-α-factor, and the images were acquired 1, 20 and 40 min after washing out unbound A594-α-factor and warming the cell to 25 °C. Scale bars, 5 μm. ( b ) Quantification of localization of A594-α-factor in wild-type and mutant cells at 20 min after internalization. Localization of A594-α-factor was categorized into three classes; vacuole only (red), endosome and vacuole (green) and endosome only (blue). Data show mean±s.d. from at least three experiments, with >100 cells counted for each strain per experiment. ( c ) Time-dependent changes of A594-α-factor localization in wild-type and vps21 Δ ypt52 Δ cells. Wild-type and vps21 Δ ypt52 Δ cells were labelled with A594-α-factor and imaged at indicated times. Scale bars, 2.5 μm. ( d ) Quantification of the number of A594-α-factor-positive endosomes displayed in ( c ). Data show the mean±s.d. of three experiments, with 50 cells counted at each time point per experiment. ( e ) Ultrastructure of endosomal compartments observed in wild-type and vps21 Δ ypt52 Δ cells. Wild-type and vps21 Δ ypt52 Δ cells were grown at 25 °C, and fixed with 2% formaldehyde and 2.5% glutaraldehyde in phosphate buffer. Arrowheads point to various sizes of vesicles that accumulate in vps21 Δ ypt52 Δ cells. V, vacuole; N, nucleus. Scale bars, 1 μm. ( f ) Immunoelectron microscopic localization of A488-α-factor in wild-type and vps21 Δ ypt52 Δ cells. Wild-type and vps21 Δ ypt52 Δ cells were incubated with A488-α-factor and internalization was induced 20 min before 4% formaldehyde/0.05% glutaraldehyde fixation. Internalized A488-α-factor was labelled with rabbit anti-Alexa Fluor 488 antibody followed by biotinylated goat anti-rabbit immunoglobulin G and then goat anti-biotin immunoglobulin G-CG (8 nm) conjugate. The bottom panel in vps21 Δ ypt52 Δ cell shows a high-magnification view of the boxed area. Arrowheads point to vesicular structures including A488-α-factor. Scale bars, 500 nm. Full size image Convergence of the endocytic pathway with the VPS pathway We next wished to investigate if VPS21 and YPT52 were required before or after the convergence of the VPS pathway with the endocytic one. We used GFP-tagged Vph1p, a vacuolar ATPase, as a marker for the VPS pathway [29] , [30] , [31] . In agreement with the previous observations [22] , Vph1p was ectopically localized to multiple punctate compartments in vps21 Δ ypt52 Δ cells ( Fig. 3a,b ). We again used A594-α-factor to mark the endocytic pathway. We found that ~70% of the Vph1-GFP in vps21 Δ ypt52 Δ cells was colocalized with A594-α-factor ( Fig. 3c,d and Supplementary Movie 3 ), supporting the conclusion that Vps21p and Ypt52p act after the convergence of the two pathways. Our results differed from previous observations that the cell surface receptor, Ste3p, and Vph1p accumulate in different transport intermediates in these cells [11] . In order to resolve this issue, we examined the localization of mCherry-fused Ste3p and Vph1-GFP in vps21 Δ ypt52 Δ cells. In wild-type cells, both Ste3p and Vph1p are transported to, and colocalized at, the vacuole ( Fig. 3e ). Unexpectedly, we observed that ~58.1% of the Vph1-GFP in vps21 Δ ypt52 Δ cells colocalized with Ste3-mCherry, in the same manner as A594-α-factor. This observation further supports the idea that the endocytic pathway intersects the VPS pathway at an early stage of endocytosis, independently of yeast Rab5s. 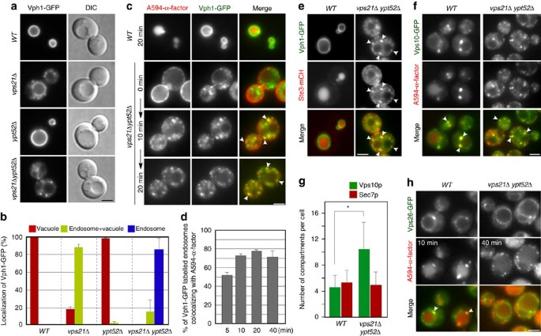Figure 3: Convergence of the endocytic pathway with the VPS pathway invps21Δypt52Δ cells. (a) Defective transport of Vph1p invps21Δypt52Δ cells. Indicated genotypes expressing Vph1-GFP were grown to early to mid-logarithmic phase in yeast extract peptone-dextrose YPD medium at 25 °C and observed by fluorescence microscopy and different interference contrast (DIC). (b) Quantification of Vph1-GFP localization in cells displayed in (a). The bar graphs represent the percentages of cells exhibiting Vph1-GFP localized at the vacuole only (red), endosome and vacuole (green) and endosome only (blue). Data show mean±s.d. from at least three experiments, with 50 cells counted for each strain per experiment. (c) Colocalization of A594-α-factor with Vph1-GFP invps21Δypt52Δ cells. A594-α-factor was added tovps21Δypt52Δ cells and followed through the endocytic pathway for the indicated times. Each image pair was acquired simultaneously at indicated time using dual-channel two-dimensional (2D) imaging system. Arrowheads indicate examples of colocalization. (d) Quantification of colocalization of A594-α-factor and Vph1-GFP invps21Δypt52Δ cells. The percentages of colocalization were calculated as the ratio of Vph1-GFP-labelled endosomes colocalizing with A594-α-factor in single focal plane images at each time point. A total of 50 Vph1-GFP-labelled endosomes were counted per experiment. Error bars represent the s.d. from at least three experiments. (e) Localization of Vph1-GFP and Ste3-mCH (mCherry) in wild-type andvps21Δypt52Δ cells. Cells expressing Vph1-GFP and Ste3-mCH were grown to early to mid-logarithmic phase and observed by dual-channel 2D fluorescence microscopy. (f) Colocalization of A594-α-factor with Vps10-GFP in wild-type andvps21Δypt52Δ cells. Cells expressing Vps10-GFP were labelled with A594-α-factor and imaged at 10 min after internalization as described in (c). Arrowheads indicate examples of colocalization. (g) Increase in the number of Vps10p positive compartments invps21Δypt52Δ cells. Cells expressing Vps10-GFP or Sec7-mCherry were grown to early to mid-logarithmic phase in YPD medium at 25 °C and observed by fluorescence microscopy. Data show mean±s.d. from at least three experiments, with 50 cells counted for each strain per experiment. Error bars represent the s.d. from at least three experiments. *P-value <0.001, unpairedt-test. (h) Simultaneous imaging of Vps26-GFP with A594-α-factor. Each image pair was acquired simultaneously at the indicated time. Arrowheads indicate examples of colocalization. Scale bars, 2.5 μm. Figure 3: Convergence of the endocytic pathway with the VPS pathway in vps21 Δ ypt52 Δ cells. ( a ) Defective transport of Vph1p in vps21 Δ ypt52 Δ cells. Indicated genotypes expressing Vph1-GFP were grown to early to mid-logarithmic phase in yeast extract peptone-dextrose YPD medium at 25 °C and observed by fluorescence microscopy and different interference contrast (DIC). ( b ) Quantification of Vph1-GFP localization in cells displayed in ( a ). The bar graphs represent the percentages of cells exhibiting Vph1-GFP localized at the vacuole only (red), endosome and vacuole (green) and endosome only (blue). Data show mean±s.d. from at least three experiments, with 50 cells counted for each strain per experiment. ( c ) Colocalization of A594-α-factor with Vph1-GFP in vps21 Δ ypt52 Δ cells. A594-α-factor was added to vps21 Δ ypt52 Δ cells and followed through the endocytic pathway for the indicated times. Each image pair was acquired simultaneously at indicated time using dual-channel two-dimensional (2D) imaging system. Arrowheads indicate examples of colocalization. ( d ) Quantification of colocalization of A594-α-factor and Vph1-GFP in vps21 Δ ypt52 Δ cells. The percentages of colocalization were calculated as the ratio of Vph1-GFP-labelled endosomes colocalizing with A594-α-factor in single focal plane images at each time point. A total of 50 Vph1-GFP-labelled endosomes were counted per experiment. Error bars represent the s.d. from at least three experiments. ( e ) Localization of Vph1-GFP and Ste3-mCH (mCherry) in wild-type and vps21 Δ ypt52 Δ cells. Cells expressing Vph1-GFP and Ste3-mCH were grown to early to mid-logarithmic phase and observed by dual-channel 2D fluorescence microscopy. ( f ) Colocalization of A594-α-factor with Vps10-GFP in wild-type and vps21 Δ ypt52 Δ cells. Cells expressing Vps10-GFP were labelled with A594-α-factor and imaged at 10 min after internalization as described in ( c ). Arrowheads indicate examples of colocalization. ( g ) Increase in the number of Vps10p positive compartments in vps21 Δ ypt52 Δ cells. Cells expressing Vps10-GFP or Sec7-mCherry were grown to early to mid-logarithmic phase in YPD medium at 25 °C and observed by fluorescence microscopy. Data show mean±s.d. from at least three experiments, with 50 cells counted for each strain per experiment. Error bars represent the s.d. from at least three experiments. * P- value <0.001, unpaired t -test. ( h ) Simultaneous imaging of Vps26-GFP with A594-α-factor. Each image pair was acquired simultaneously at the indicated time. Arrowheads indicate examples of colocalization. Scale bars, 2.5 μm. Full size image Similar to the effect on A594-α-factor ( Fig. 2a,b ), Vph1-GFP localized normally to the vacuole in ypt52 Δ mutants, whereas the combination of the vps21 Δ and ypt52 Δ mutations showed a more severe phenotype, blocking Vph1p transport beyond the endosome ( Fig. 3a,b ) with ~85% of cells now showing localization only to the endosome and not the vacuole. These data suggested that convergence of the endocytic pathway with the VPS pathway is not impaired in vps21 Δ ypt52 Δ cells and that they work together to permit transport from the endosome to the vacuole. To confirm this finding, we also used another marker for the VPS pathway, Vps10p, which is reported to cycle between the TGN and prevacuolar/late endosomal compartments through the early endosome [3] , [32] , [33] . Similarly to Vph1p, Vps10p accumulated in prevalent punctate compartments labelled with A594-α-factor in vps21 Δ ypt52 Δ cells ( Fig. 3f,g ). In contrast, we found that A594-α-factor rarely colocalized with the late endosomal/prevacuolar compartment marker Vps26p in vps21 Δ ypt52 Δ cells ( Fig. 3h ) [25] , [26] . Since most of the A594-α-factor was transported to the vacuole through Vps26p-positive compartments that were highly colocalized with Vps21p in wild-type cells ( Figs 1e and 3h ), it seems that A594-α-factor was unable to reach the late endosomal/PVCs in vps21 Δ ypt52 Δ cells. Collectively, our results suggest that Vps21p and Ypt52p are not required for the fusion of endocytic vesicles with TGN-derived transport vesicles utilizing the VPS pathway, but are essential for progression of cargo beyond early endosomes. Involvement of the AP-3 pathway in the endocytic pathway Transport of A594-α-factor to the vacuole was retarded but not completely blocked in vps21 Δ ypt52 Δ and vps21 Δ ypt52 Δ ypt53 Δ mutants ( Figs 2b and 4a,b ). Therefore, we speculated that α-factor might bypass the transport defect in these mutants by utilizing other intracellular trafficking pathway(s) en route to the vacuole. The AP-3 complex-mediated pathway is known to be another pathway for transporting biosynthetic cargo from the TGN to the vacuole in most eukaryotic cells [34] . We first examined if the AP-3 pathway was still intact upon deletion of VPS21 family genes, using the chimeric protein GFP–Nyv1–Snc1-TMD (GNS), which accumulates at the plasma membrane if the AP-3 pathway is defective [35] . While GNS was missorted to the plasma membrane in cells depleted of Apm3p, it was transported normally in vps21 Δ ypt52 Δ or vps21 Δ ypt52 Δ ypt53 Δ mutants ( Fig. 4c ), indicating the presence of a functional AP-3 pathway capable of transporting cargos from the TGN to the vacuole. To examine the involvement of the AP-3 pathway in α-factor transport in Rab5 -disrupted cells, we further deleted the APM3 gene in vps21 Δ ypt52 Δ ypt53 Δ mutants. Since the vacuoles in the vps21 Δ ypt52 Δ ypt53 Δ apm3 Δ quadruple mutant appeared to be smaller than those in other mutants, we assessed the integrity of the vacuoles in each mutant. As reported previously, vps21 Δ ypt52 Δ and vps21 Δ ypt52 Δ ypt53 Δ cells exhibited a class D-like vps phenotype, characterized by vacuolar enlargement, similar to that reported for vps21 Δ cells ( Supplementary Fig. 3a ) [22] , [31] . By using different interference contrast microscopy, we observed that most of the wild-type, vps21 Δ, vps21 Δ ypt52 Δ or vps21 Δ ypt52 Δ ypt53 Δ cells contained single or multiple vacuoles ( Supplementary Fig. 3a,b ). In contrast, the proportion of quadruple mutant cells containing visible vacuoles was decreased to ~78.8% ( Supplementary Fig. 3a,b ). These results suggest that the AP-3-mediated pathway might be required for transporting membrane lipids, as well as cargo proteins, to the vacuole from the Golgi in Rab5 -disrupted cells. We next examined A594-α-factor transport to the vacuole in these mutants in the majority of cells that contained visible vacuole(s). Intriguingly, we found that α-factor transport was little affected by the apm3 Δ mutant but severely affected in the quadruple mutant ( Fig. 4a,b ). We also found that α-factor transport in vps21 Δ apm3 Δ cells is slightly delayed, compared with that in vps21 Δ single mutant cells ( Supplementary Fig. 3c ), suggesting that α-factor is transported to the vacuole via the AP-3-mediated pathway in Rab5 -disrupted cells. 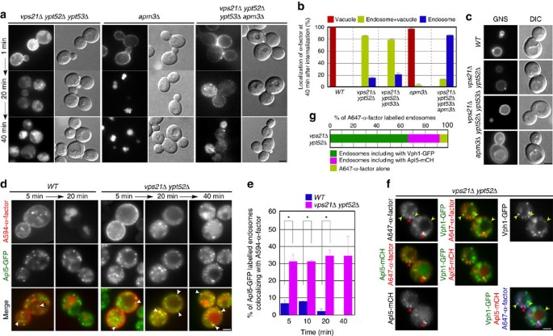Figure 4: Involvement of the AP-3-mediated pathway in A594-α-factor delivery to vacuole. (a) Defective transport of A594-α-factor invps21Δypt52Δypt53Δ cells is enhanced inapm3Δ. A594-α-factor was allowed to bind tovps21Δypt52Δypt53Δ,apm3Δ cells orvps21Δypt52Δypt53Δapm3Δ cells, and its localization was followed for the indicated times. (b) Quantification of A594-α-factor localization in cells displayed in (a). Localization of A594-α-factor was analysed at 40 min after internalization, and categorized into three classes; endosome only (blue), endosome and vacuole (green) and vacuole only (red). Data show mean±s.d. from at least three experiments, with >100 cells counted for each strain per experiment. (c) Analysis of the AP-3 pathway in wild-type and mutant cells. Cells expressing GFP–Nyv1–Snc1-TMD (GNS) fusion protein were grown to early to mid-logarithmic phase at 25 °C and observed by fluorescence microscopy and different interference contrast (DIC). (d) Partial colocalization of Apl5-GFP with A594-α-factor in wild-type andvps21Δypt52Δ cells. A594-α-factor was added to wild-type orvps21Δypt52Δ cells and followed through the endocytic pathway for the indicated times. Each image pair was acquired simultaneously at the indicated time using dual-channel 2D imaging system. Arrowheads indicate examples of colocalization. (e) Quantification of colocalization of A594-α-factor with Apl5-GFP in wild-type andvps21Δypt52Δ cells. The histogram shows the percentages of Apl5-GFP-labelled endosomes colocalizing with A594-α-factor. The percentages of colocalization were calculated using single focal plane images. Greater than 100 Apl5-GFP-labelled endosomes were counted at each time point per experiment. Error bars represent the s.d. from at least three experiments. *P-value <0.001, unpairedt-test. (f) Internalized A647-α-factor resides both in the VPS and the AP-3 pathway.vps21Δypt52Δ cells expressing Vph1-GFP and Apl5-mCH (mCherry) were incubated with A647-α-factor and internalization was induced for 20 min prior to imaging. Each image pair was acquired using fluorescence microscopy equipped with a high-speed filter changer. Time to acquire one image pair is 3.5 s. Arrowheads indicate examples of colocalization between Vph1-GFP and A647-α-factor (yellow arrowheads) or Apl5-mCH and A647-α-factor (red arrowheads). (g) Quantification of colocalization of A647-α-factor with Vph1-GFP (dark green), or Apl5-mCherry (magenta) shown inFig. 4f. The percentages of colocalization were calculated using single focal plane images. Data show the mean of three experiments, with >50 A647-α-factor-labelled endosomes counted per experiment. Scale bars, 2.5 μm. Figure 4: Involvement of the AP-3-mediated pathway in A594-α-factor delivery to vacuole. ( a ) Defective transport of A594-α-factor in vps21 Δ ypt52 Δ ypt53 Δ cells is enhanced in apm3 Δ. A594-α-factor was allowed to bind to vps21 Δ ypt52 Δ ypt53 Δ, apm3 Δ cells or vps21 Δ ypt52 Δ ypt53 Δ apm3 Δ cells, and its localization was followed for the indicated times. ( b ) Quantification of A594-α-factor localization in cells displayed in ( a ). Localization of A594-α-factor was analysed at 40 min after internalization, and categorized into three classes; endosome only (blue), endosome and vacuole (green) and vacuole only (red). Data show mean±s.d. from at least three experiments, with >100 cells counted for each strain per experiment. ( c ) Analysis of the AP-3 pathway in wild-type and mutant cells. Cells expressing GFP–Nyv1–Snc1-TMD (GNS) fusion protein were grown to early to mid-logarithmic phase at 25 °C and observed by fluorescence microscopy and different interference contrast (DIC). ( d ) Partial colocalization of Apl5-GFP with A594-α-factor in wild-type and vps21 Δ ypt52 Δ cells. A594-α-factor was added to wild-type or vps21 Δ ypt52 Δ cells and followed through the endocytic pathway for the indicated times. Each image pair was acquired simultaneously at the indicated time using dual-channel 2D imaging system. Arrowheads indicate examples of colocalization. ( e ) Quantification of colocalization of A594-α-factor with Apl5-GFP in wild-type and vps21 Δ ypt52 Δ cells. The histogram shows the percentages of Apl5-GFP-labelled endosomes colocalizing with A594-α-factor. The percentages of colocalization were calculated using single focal plane images. Greater than 100 Apl5-GFP-labelled endosomes were counted at each time point per experiment. Error bars represent the s.d. from at least three experiments. * P- value <0.001, unpaired t -test. ( f ) Internalized A647-α-factor resides both in the VPS and the AP-3 pathway. vps21 Δ ypt52 Δ cells expressing Vph1-GFP and Apl5-mCH (mCherry) were incubated with A647-α-factor and internalization was induced for 20 min prior to imaging. Each image pair was acquired using fluorescence microscopy equipped with a high-speed filter changer. Time to acquire one image pair is 3.5 s. Arrowheads indicate examples of colocalization between Vph1-GFP and A647-α-factor (yellow arrowheads) or Apl5-mCH and A647-α-factor (red arrowheads). ( g ) Quantification of colocalization of A647-α-factor with Vph1-GFP (dark green), or Apl5-mCherry (magenta) shown in Fig. 4f . The percentages of colocalization were calculated using single focal plane images. Data show the mean of three experiments, with >50 A647-α-factor-labelled endosomes counted per experiment. Scale bars, 2.5 μm. Full size image We next sought direct evidence that A594-α-factor could be transported to the vacuole via the AP-3 pathway, independently of the VPS pathway. We utilized A594-α-factor and GFP-fused Apl5p, an AP-3 complex subunit localizing at the TGN and transport vesicles [36] . Apl5-GFP was observed in the cytoplasm as multiple small puncta, and the localization and number of Apl5-GFP puncta were not affected by deleting yeast Rab5s or expressing mCherry-tagged Abp1p ( Supplementary Fig. 4 and Supplementary Movie 4 ). We found that a proportion of the A594-α-factor became transiently colocalized with Alp5p-residing vesicles and was then translocated to the vacuole, in both wild-type and vps21 Δ ypt52 Δ cells, although the trafficking was retarded in vps21 Δ ypt52 Δ cells relative to wild-type cells ( Fig. 4d,e ). Approximately 80% of Apl5p appeared to reside on vesicles that do not include Vph1p in vps21 Δ ypt52 Δ cells ( Supplementary Fig. 5a ) supporting the idea that the VPS and AP-3 pathway are separate. About 20% of each of the Vph1p and Apl5p localization also colocalized with Sec7p, suggesting that colocalization of Apl5p and Vph1p occurred predominantly at the TGN in vps21 Δ ypt52 Δ cell ( Supplementary Fig. 5a–c ). Again, neither Vph1p nor Apl5p colocalized with the mitochondria labelled by mitotracker (<2%) used as a negative control ( Supplementary Fig. 5d ). Furthermore, triple staining of vps21 Δ ypt52 Δ cells with Vph1-GFP, Apl5-mCherry and Alexa Fluor 647-labelled α-factor (A647-α-factor) demonstrated that ~65.3% and ~26.6% of α-factor resided in the VPS pathway and the AP-3 pathway, respectively, on different endosomes ( Fig. 4f,g ). Although triple colour imaging causes a ~2.5-s time lag for acquiring three different colour images, we detected remarkable colocalization of α-factor with Vph1p or Apl5p in distinct endosomes in vps21 Δ ypt52 Δ cell. This could be due to the relatively slow motility of endosomes accumulated in vps21 Δ ypt52 Δ cell. As shown in Supplementary Movie 3 , endosomes containing both α-factor and Vph1p at 20 min after α-factor internalization often stay around more than several seconds and therefore made it easy to observe colocalization. We hypothesize that the motility of endosomes might decrease in vps21 Δ ypt52 Δ cells because the fusion or maturation of these endosomes is suppressed. The AP-3-mediated endocytic pathway exists in wild-type cells We next investigated the AP-3-mediated endocytic pathway in wild-type cells. As shown in Fig. 5a,b , Vps21p colocalized little with Apl5p (~5.4%), and A647-α-factor was located in distinct Apl5p- or Vps21p-labelled endosomes in wild-type cells, supporting the idea that the AP-3-mediated endocytic pathway is independent of Rab5. Although colocalization of α-factor with Apl5p or Vps21p was detected by triple staining ( Fig. 5b ), since some of the endosomes in which α-factor resides in wild-type cells move actively and fuse with each other at 5–10 min after α-factor internalization ( Fig. 1g and Supplementary Movie 1 ), it was a little inaccurate to quantify colocalization between these molecules by using triple staining which has a ~2.5 s lag for acquisition of all three channels. To assess with high precision what % of α-factor is transported via the Rab5-independent AP-3 pathway in wild-type cell, we analysed colocalization between A594-α-factor and Vps21p or Apl5p by simultaneous double colour time-lapse imaging. Live-cell imaging of Apl5-GFP and A594-α-factor demonstrated that appreciable localization of A594-α-factor was observed in several Apl5-GFP-labelled endosomes in wild-type cells ( Fig. 5c,d and Supplementary Movie 5 ). To quantify the colocalization accurately, we defined the colocalization by the presence of two fluorescence molecules at the same endosome for at least 5 s in the time-lapse imaging. These analyses demonstrated that ~11.1% or ~82.6% of A594-α-factor resides in and moves together with Apl5-GFP or GFP-Vps21p ( Supplementary Movie 1 ), respectively ( Fig. 5e ). These results, taken together, suggest the presence of a novel AP-3-mediated endocytic pathway en route to the vacuole in wild-type cells. 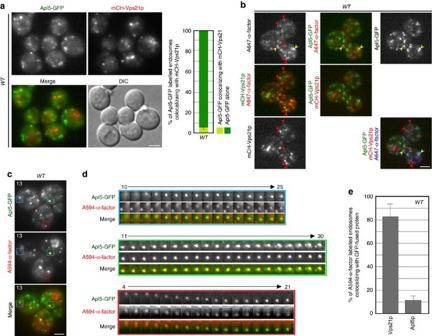Figure 5: The Rab5-independent AP-3-mediated endocytic pathway in wild-type cell. (a) Distinct localization pattern of Apl5p and Vps21p in wild-type cells. Each image pair was acquired simultaneously using a dual-channel imaging system. Quantification of colocalization is shown on the right. Data show mean±s.d. from at least three experiments, with 100 Apl5-GFP-labelled endosomes counted per experiment. The percentages of colocalization were calculated using single focal plane images. (b) Internalized A647-α-factor resides in distinct Apl5p- or Vps21p-labelled endosomes. Wild-type cells expressing mCH (mCherry)-Vps21 and Apl5-GFP were incubated with A647-α-factor and internalization was induced for 5 min prior to imaging. Each image pair was acquired using fluorescence microscopy equipped with a high-speed filter changer. Arrowheads indicate examples of colocalization of Apl5-GFP and A647-α-factor (yellow arrowheads) or mCH-Vps21and A647-α-factor (red arrowheads). Time to acquire one image pair is 3.5 s. (c,d) Dynamic behaviour of endosomes on which both A594-α-factor and Apl5p reside in wild-type cells. (c) Single frames (frame 13) fromSupplementary Movie 5of wild-type cells showing GFP (Apl5) and mCherry (α-factor) channels, and a merged image. Each image pair was simultaneously acquired at successive 1-s intervals using a dual-channel two-dimensional (2D) imaging system. (d) Time series of single patches in the boxed area in (c). Upper panels (10–25 s) correspond to the area boxed in blue in (c), middle panels (11–30 s) correspond to area boxed in green in (c), and lower panels (4–21 s) correspond to area boxed in red in (c), respectively. (e) Quantification of colocalization of A594-α-factor with GFP-Vps21p or Apl5-GFP in wild-type cells. The histogram shows the percentages of A594-α-factor-labelled endosomes colocalizing with GFP-fused proteins. Colocalization was defined by the presence of two fluorescence molecules at the same location for at least five frames (>5 s) in the time-lapse imaging acquired by simultaneous dual-channel 2D imaging system. Data show the mean±s.d. of three experiments, with >50 A594-α-factor-labelled endosomes counted per experiment. Scale bars, 2.5 μm. Figure 5: The Rab5-independent AP-3-mediated endocytic pathway in wild-type cell. ( a ) Distinct localization pattern of Apl5p and Vps21p in wild-type cells. Each image pair was acquired simultaneously using a dual-channel imaging system. Quantification of colocalization is shown on the right. Data show mean±s.d. from at least three experiments, with 100 Apl5-GFP-labelled endosomes counted per experiment. The percentages of colocalization were calculated using single focal plane images. ( b ) Internalized A647-α-factor resides in distinct Apl5p- or Vps21p-labelled endosomes. Wild-type cells expressing mCH (mCherry)-Vps21 and Apl5-GFP were incubated with A647-α-factor and internalization was induced for 5 min prior to imaging. Each image pair was acquired using fluorescence microscopy equipped with a high-speed filter changer. Arrowheads indicate examples of colocalization of Apl5-GFP and A647-α-factor (yellow arrowheads) or mCH-Vps21and A647-α-factor (red arrowheads). Time to acquire one image pair is 3.5 s. ( c , d ) Dynamic behaviour of endosomes on which both A594-α-factor and Apl5p reside in wild-type cells. ( c ) Single frames (frame 13) from Supplementary Movie 5 of wild-type cells showing GFP (Apl5) and mCherry (α-factor) channels, and a merged image. Each image pair was simultaneously acquired at successive 1-s intervals using a dual-channel two-dimensional (2D) imaging system. ( d ) Time series of single patches in the boxed area in ( c ). Upper panels (10–25 s) correspond to the area boxed in blue in ( c ), middle panels (11–30 s) correspond to area boxed in green in ( c ), and lower panels (4–21 s) correspond to area boxed in red in ( c ), respectively. ( e ) Quantification of colocalization of A594-α-factor with GFP-Vps21p or Apl5-GFP in wild-type cells. The histogram shows the percentages of A594-α-factor-labelled endosomes colocalizing with GFP-fused proteins. Colocalization was defined by the presence of two fluorescence molecules at the same location for at least five frames (>5 s) in the time-lapse imaging acquired by simultaneous dual-channel 2D imaging system. Data show the mean±s.d. of three experiments, with >50 A594-α-factor-labelled endosomes counted per experiment. Scale bars, 2.5 μm. Full size image Association of endocytic vesicles with AP-3-coated vesicles The unexpected connection between endocytic trafficking and the AP-3 pathway motivated us to further examine the dynamics of endocytic vesicles and Apl5p-residing endosomes in vps21 Δ ypt52 Δ cells. Abp1p is a marker used for visualizing the formation and internalization of endocytic vesicles [37] , and we previously showed that after binding to α-factor, the Ste2p receptor is recruited to and endocytosed via Abp1p-labelled clathrin-coated vesicles [23] , [28] . Accordingly, we considered Abp1-mCherry patches to be endocytic vesicles in which α-factor and its receptor would be incorporated, and analysed their dynamics in vps21 Δ ypt52 Δ cells. The lifetime of Abp1-mCherry patches in vps21 Δ ypt52 Δ cells (14.7±2.9 s, mean±s.d., n =50 patches) was almost the same as that in wild-type cells (14.2±2.1 s, n =50 patches) ( Fig. 6a ). The fluorescence intensity and inward movement of Abp1-mCherry patches in vps21 Δ ypt52 Δ cells were also similar to those in wild-type cells ( Fig. 6b,c ), indicating that formation and internalization of endocytic vesicles at the plasma membrane appeared to be normal. Interestingly, by colabelling with Abp1p and Apl5p, we observed that some endocytic vesicles, moving in a directed manner toward Apl5p-positive endosomes, become transiently colocalized and move with Apl5p-positive endosomes before disappearing in vps21 Δ ypt52 Δ cells ( Fig. 6d,e and Supplementary Movie 6 ). Quantitative analyses revealed that ~30% of Abp1p-labelled endocytic vesicles showed such dynamics both in wild-type and vps21 Δ ypt52 Δ cells ( Fig. 6f ). Thus, in yeast, endocytic vesicles appear to associate directly with TGN-derived transport vesicles in the AP-3 pathway, independently of Rab5. To exclude the possibility that α-factor is first transported to the early or late Golgi and then exits via the VPS or AP-3 pathway, we examined whether A594-α-factor passes through the early/late Golgi en route to the vacuole. Vrg4p, an early Golgi marker, and Sec7p, a late Golgi marker, showed distinct distribution patterns, and less than 5% of these proteins were colocalized ( Supplementary Fig. 6a ). As shown in Supplementary Fig. 6b–d , A594-α-factor colocalized with neither Sec7p nor Vrg4p in wild-type cells at any of the time points examined. This suggests that transport of α-factor from the plasma membrane to the vacuole is not mediated via the Golgi compartments. 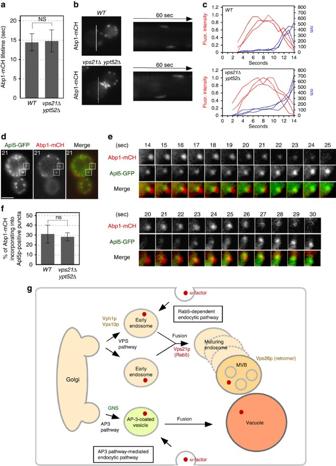Figure 6: Dynamic behavior of endosomes and endocytic vesicles in the AP-3 pathway. (a) Average lifetimes of Abp1-mCH (mCherry)±s.d. in wild-type andvps21Δypt52Δ cells. Data were taken from 1-min movie with a 1-s frame interval.n=50 patches for each strain. NS: non-statistically significant (P-value >0.5, unpairedt-test). (b) Localization of Abp1-mCherry in wild-type andvps21Δypt52Δ cells (left panels). Lines in the image mark where the kymograph in right-hand panels was generated. (c) Quantification of fluorescence intensity (red) and distance from the site of patch formation (blue) as a function of time for Abp1-mCherry patches. Each curve represents data from one patch. Behaviour of three independent patches was plotted for each strain. All movies were taken with a 1-s frame interval. (d,e) Movement of Abp1-mCherry patches towards Apl5p-positive endosomes. (d) Single frames from movies ofvps21Δypt52Δ cells showing the GFP and the mCherry channels, and a merged image. Each image pair was acquired simultaneously using dual-channel time-lapse imaging system. Scale bars, 2.5 μm. (e) Time series of single patches in boxed area in (d). Upper panels (14–25 s) correspond to upper boxed area in (d), and lower panels (20–30 s) correspond to lower boxed area in (d), respectively. (f) Quantification of incorporation of Abp1-mCH into Apl5-GFP in wild-type andvps21Δypt52Δ cells. The histogram shows the percentages of Abp1-mCH incorporating into Apl5p-positive puncta. Greater than 50 Abp1-mCH-labelled patches were counted for each strain per experiment. Error bars represent the s.d. from at least three experiments. NS: non-statistically significant (P-value >0.5, unpairedt-test). (g) Model of two distinct endocytic pathways. Vps21p functions in a Rab5-dependent endocytic pathway that intersects with the VPS pathway, but not in another endocytic pathway mediated by the AP-3 adaptor complex. Figure 6: Dynamic behavior of endosomes and endocytic vesicles in the AP-3 pathway. ( a ) Average lifetimes of Abp1-mCH (mCherry)±s.d. in wild-type and vps21 Δ ypt52 Δ cells. Data were taken from 1-min movie with a 1-s frame interval. n =50 patches for each strain. NS: non-statistically significant ( P- value >0.5, unpaired t -test). ( b ) Localization of Abp1-mCherry in wild-type and vps21 Δ ypt52 Δ cells (left panels). Lines in the image mark where the kymograph in right-hand panels was generated. ( c ) Quantification of fluorescence intensity (red) and distance from the site of patch formation (blue) as a function of time for Abp1-mCherry patches. Each curve represents data from one patch. Behaviour of three independent patches was plotted for each strain. All movies were taken with a 1-s frame interval. ( d , e ) Movement of Abp1-mCherry patches towards Apl5p-positive endosomes. ( d ) Single frames from movies of vps21 Δ ypt52 Δ cells showing the GFP and the mCherry channels, and a merged image. Each image pair was acquired simultaneously using dual-channel time-lapse imaging system. Scale bars, 2.5 μm. ( e ) Time series of single patches in boxed area in ( d ). Upper panels (14–25 s) correspond to upper boxed area in ( d ), and lower panels (20–30 s) correspond to lower boxed area in ( d ), respectively. ( f ) Quantification of incorporation of Abp1-mCH into Apl5-GFP in wild-type and vps21 Δ ypt52 Δ cells. The histogram shows the percentages of Abp1-mCH incorporating into Apl5p-positive puncta. Greater than 50 Abp1-mCH-labelled patches were counted for each strain per experiment. Error bars represent the s.d. from at least three experiments. NS: non-statistically significant ( P- value >0.5, unpaired t -test). ( g ) Model of two distinct endocytic pathways. Vps21p functions in a Rab5-dependent endocytic pathway that intersects with the VPS pathway, but not in another endocytic pathway mediated by the AP-3 adaptor complex. Full size image On the basis of the data presented above and in previous studies, we propose that the endocytic pathway separately intersects with two vacuolar-targeting pathways: the Rab5-dependent VPS pathway and the Rab5-independent AP-3-mediated direct trafficking pathway ( Fig. 6g ). We also demonstrate that convergence of the endocytic and VPS pathways can occur at an early stage of endocytosis, independently of Rab5. Several studies based on FM4-64 uptake experiments and colocalization with TGN markers in higher plants and yeast have indicated that the TGN itself, or an intermediate TGN derivative, acts as an early endosome, receiving endocytosed material from the plasma membrane [38] , [39] , [40] , [41] . In previous studies using tobacco BY-2 cells, Jiang and his colleagues [39] demonstrated that FM4-64 internalized from the plasma membrane reaches early/recycling endosomes, which are characteristic clathrin-coated TGN compartments defined by SCAMP1 and V-ATPase, before reaching the PVC/MVB [39] , [42] . This finding suggests that a trafficking pathway exists that is conserved between yeast and plants, although whether the TGN compartment serves as an early/recycling endosome remains unclear. FM4-64 is an excellent marker of the endocytic pathway in a broad range of organisms, but there is still some debate about the precise pathways of intracellular transport it follows, as FM4-64 is known to be distributed to different organelle membranes after endocytic internalization. In plant cells, FM4-64 becomes localized to the Golgi, PVC and vacuolar membrane after 30 min of staining, and to many organelles involved in the secretory and recycling pathways, as well as the endocytic pathway, by 60 min (ref. 43 ). In yeast, secretion of endocytosed FM4-64 via the recycling pathway is more rapid, and around half of the endocytosed FM4-64 is secreted within 10 min via the recycling pathway [44] , probably through the TGN compartments. These observations suggest that it would be difficult to determine whether the FM4-64 fluorescence at the TGN seen by Jiang and colleagues [39] is directly derived from the plasma membrane via the endocytic pathway or from the early/recycling endosome via the recycling pathway. In contrast, fluorescence labelling of α-factor labels the endocytic pathway specifically and time dependently, and does not label other pathways such as the recycling pathway, thereby allowing visualization of the whole route taken by endocytosed cargo before delivery to the vacuole. In this study, we demonstrated that A594-α-factor-containing endosomes intersect the VPS pathway at post-TGN vesicles, not the TGN, since endocytosed A594-α-factor was not accessible to Sec7p-residing TGN ( Supplementary Fig. 6b ). Thus, in yeast, endocytic compartments that converge on the VPS pathway are likely to be neither TGN nor PVC/MVB. In contrast to a previous observation [11] , we demonstrated that Ste3p and Vph1p reside in the same intracellular compartments in vps21 Δ ypt52 Δ cells. Gerrard et al. [11] separated the P13 membrane fraction of vps21 Δ mutants by sucrose density gradient fractionation, and observed that Vph1p and Ste3p were separated in different subcellular fractions, suggesting that Ste3p and Vph1p do not accumulate in the same trafficking intermediates in vps21 Δ cells [11] . However, they also showed that both Ste3p and Vph1p separated in the P100 fraction, which includes Golgi membranes and transport vesicles, although they did not examine the P100 fraction itself [11] . Thus, Ste3p and Vph1p might accumulate in the same transport vesicles that are included in the P100 fraction. The location where AP-3 function is required has been unclear. Similarly to what is seen for the yeast AP-3 complex, loss of a functional AP-3 complex in mammalian cells leads to defects in the trafficking of several lysosomal membrane proteins, such as LAMPs and CD63, to the plasma membrane [45] , [46] . A previous electron microscopy analysis in NRK cells demonstrated that AP-3 labelling is mainly associated within the TGN [47] , indicating the similar role of AP-3 in the intracellular transport from the TGN to lysosome. By contrast, several studies demonstrate the role of AP-3 complex at early endosomal compartments. A quantitative study of AP-3 localization in HepG2 cells has revealed that AP-3-positive buds reside on the tubular recycling endosomes evolving from early endosomes that contain internalized transferrin and cation-independent mannose 6-phosphate receptor, markers of the endocytic recycling pathway [12] . It is also reported that endocytosed VAMP7, a SNARE involved in the fusion of late endosomes and lysosomes, binds the δ-adaptin subunit of the AP-3 complex at the early endosome, and then is transported to the late endosome/lysosomal compartment [13] . Whether AP-3 functions at early endosomal compartments, as shown in mammalian cells, or at the TGN, as originally proposed for yeast, is still under debate. Our findings provide an answer for this issue. AP-3 complex is first recruited to the TGN and forms vesicles containing lysosomal proteins. The AP-3-coated vesicle then fuses to endocytic vesicles, resulting in the formation of the early endocytic compartment ( Fig. 6g ). Thus, the AP-3 complex can function both at TGN and early endocytic compartment. Yeast strains and plasmids The yeast strains used in this study are listed in Supplementary Table 1 . All strains were grown in standard rich medium (YPD) or synthetic medium (SM) supplemented with 2% glucose and appropriate amino acids. The amino-terminal GFP tag was integrated at the endogenous locus of the VPS21 gene as follows: The GFP (S65T) fragment whose stop codon was replaced with BglII site was subcloned into BamHI- and NotI-digested pBlueScript II SK (pBS-GFP), and the Not I- Sac II fragment, which contains the S. cerevisiae ADH1 terminator and the His3MX6 module, was amplified by PCR using pFA6a-GFP (S65T)-HIS3MX6 as a template, and inserted into Not I- and Sac II-digested pBS-GFP (pBS-GFP-HIS3). To create an integration plasmid, 245-bp 5′ UTR of VPS21 gene and the N-terminal fragment of the VPS21 ORF (nt 1-476) were generated by PCR and cloned into the BamHI or BglII site of pBS-GFP-HIS3 (see Supplementary Fig. 1a ). To integrate GFP at the N terminus of the VPS21 gene, the integration plasmid was linearized by EcoRV and transformed into yeast. The extra region generated by insertion of the integration plasmid was removed by PCR-based homologous recombination as shown in Supplementary Fig. 1a . The carboxy-terminal GFP or mCherry tagging of proteins was performed by PCR-based homologous recombination using pFA6a-GFP(S65T) or pFA6a-mCherry, respectively, as a template [48] . Fluorescence microscopy Fluorescence microscopy was performed using an Olympus IX81 microscope equipped with a × 100/NA 1.40 (Olympus) objective and Orca-AG cooled CCD camera (Hamamatsu), using Metamorph software (Universal Imaging). Simultaneous imaging of red and green fluorescence was performed using an Olympus IX81 microscope, described above, and an image splitter (Dual-View; Optical Insights) that divided the red and green components of the images with a 565-nm dichroic mirror and passed the red component through a 630/50 nm filter and the green component through a 530/30 nm filter. These split signals were taken simultaneously with one CCD camera, described above. To show what % of colocalization using the method is seen with a marker that is really in a distinct compartment, mitotracker (Life Technologies), a marker for mitochondria, was used as a negative control. Triple colour imaging of GFP, mCherry and Alexa Fluor 647 was performed using an Olympus IX81 microscope equipped with a high-speed filter changer (Lambda 10-3; Shutter Instruments) that can change filter sets within 40 ms. Fluorescence labelling of α-factor and endocytosis assays 3-Thiopropionyl-G 3 was appended to the free ∈ -amine of K 7 in otherwise fully protected α-factor by standard DCC/HOBT FMOC solid phase chemistry, and Alexa-594 maleimide (Life technologies) was coupled to the purified peptide in NMM-HOAc buffer, pH 8.0. Peptides were purified by reversed-phase HPLC; structure and purity (>97%) were assessed by ESI-FTICR mass spectrometry (Bruker, 9.4T). For endocytosis assays, cells were grown to an OD 600 of ~0.5 in 0.5 ml YPD, briefly centrifuged and resuspended in 20 μl SM with 5 μM Alexa Fluor-labelled α-factor. After incubation on ice for 2 h, the cells were washed with ice-cold SM. Internalization was initiated by addition of SM containing 4% glucose and amino acids at 25 °C. Electron microscopy For morphological observation, chemically fixed specimens were embedded in Epoxy resin, and ultrathin sections were contrasted with 2% uranyl acetate in 70% methanol and Reynolds’ lead citrate. For immunoelectron microscopy, ultrathin sections of Lowicryl K4M-embedded specimens were treated with 5% NHS/1% bovine serum albumin in phosphate-buffered saline (PBS) for 10 min to block non-specific binding, and then incubated with polyclonal rabbit anti-Alexa 488 (Invitrogen) at 4 °C overnight. After washing with PBS, the sections were incubated with biotinylated goat anti-rabbit immunoglobulin G (Vector Laboratories) at RT for 40 min. After washing with PBS, the sections were incubated with goat anti-biotin immunoglobulin G conjugated with 8 nm colloidal gold at RT for 30 min. After washing with distilled water and drying, the sections were contrasted and observed in a transmission electron microscope (1200EX; JEOL) operating at 80 kV. How to cite this article : Toshima, J. Y. et al. Bifurcation of the endocytic pathway into Rab5-dependent and -independent transport to the vacuole. Nat. Commun. 5:3498 doi: 10.1038/ncomms4498 (2014).